Bimodal magmatism produced by progressively inhibited crustal assimilation The origin of bimodal (mafic–felsic) rock suites is a fundamental question in volcanology. Here we use major and trace elements, high-resolution Sr, Nd and Pb isotope analyses, experimental petrology and thermodynamic modelling to investigate bimodal magmatism at the iconic Carlingford Igneous Centre, Ireland. We show that early microgranites are the result of extensive assimilation of trace element-enriched partial melts of local metasiltstones into mafic parent magmas. Melting experiments reveal the crust is very fusible, but thermodynamic modelling indicates repeated heating events rapidly lower its melt-production capacity. Granite generation ceased once enriched partial melts could no longer form and subsequent magmatism incorporated less fertile restite compositions only, producing mafic intrusions and a pronounced compositional gap. Considering the frequency of bimodal magma suites in the North Atlantic Igneous Province, and the ubiquity of suitable crustal compositions, we propose ‘progressively inhibited crustal assimilation’ (PICA) as a major cause of bimodality in continental volcanism. The processes that cause bimodal volcanic suites have been the subject of much debate since bimodality was first recognized some 160 years ago [1] . Volcanic and magmatic bimodality, also known as the Bunsen–Daly Gap [1] , [2] , is recognized in a variety of tectonic settings and potential explanations range from liquid immiscibility and deep trapping of intermediate magmas, to chemical interaction with crustal rocks [3] , [4] , [5] , [6] , [7] , [8] , but as yet no consensus exists. Recent advances in thermodynamic and numerical modelling support the generation of felsic magmas by crustal melting during the intrusion of basalt [9] , [10] , [11] , [12] , particularly in regions with thickened continental crust. Large mafic igneous provinces (LIPs) frequently include a significant component of silicic rocks, often in a bimodal (mafic–felsic) distribution [13] . The North Atlantic Igneous Province (NAIP) is one such LIP [13] , and formed in response to the opening of the North Atlantic Ocean (62–54 Myr ago) [14] ( Fig. 1a ). The associated pre-breakup continental magmatism includes the British–Irish Palaeogene Igneous Province (BPIP) (62–56 Myr ago), where mantle-derived magmas traversed a relatively thick, fusible continental crust [15] , [16] . Notably, almost all BPIP intrusive centres are bimodal with characteristic gabbro–granite associations (including Skye, Rum, Ardnamurchan, Mull, Slieve Gullion and Carlingford), and frequently show intense mingling and mixing between these end-member compositions [15] , [17] , [18] , [19] . The co-occurrence of mafic and felsic magmas has been proposed to be the result of incomplete mixing in compositionally stratified magma chambers [20] and suggests a rapid return to mafic magmatism once felsic magmas have been generated. Mafic replenishments into felsic magma reservoirs are considered an important trigger for large caldera-forming events in the North Atlantic Igneous Province and elsewhere (for example, Rum [21] , Skye [18] , Askja [18] and perhaps Carlingford [22] ) and can therefore fundamentally alter the eruptive style and behaviour of a volcanic system. 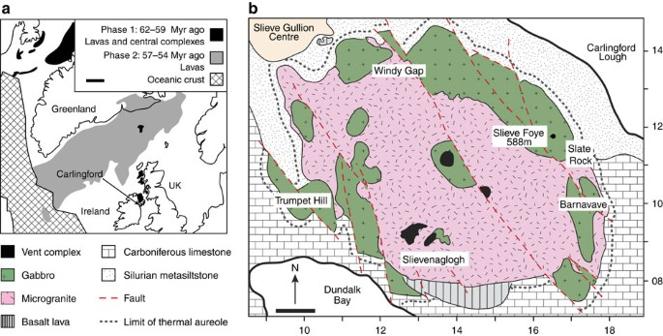Figure 1: Regional location and bedrock geology of the Carlingford Igneous Centre. (a) End-Paleocene reconstruction of the North Atlantic Igneous Province. Scale bar, 200 km. Adapted with permission from Fig. 7, Saunderset al.14, Chemical Geology, v. 241, issues 3–4, Regional uplift associated with continental large igneous provinces: The role of mantle plumes and the lithosphere, 282–318, Elsevier (2007). (b) Map of the Carlingford Igneous Centre, showing the Irish National Grid. Cone-sheet intrusions not shown. A thermal aureole of 100–200 m thickness surrounds the igneous centre. Scale bar, 1 km. Intrusions of the adjacent Slieve Gullion Igneous Centre are shown in yellow. Reproduced with permission from the Geological Survey of Ireland 1:100,000 scale bedrock geology map, Geological Survey of Ireland/Government of Ireland (2014). Figure 1: Regional location and bedrock geology of the Carlingford Igneous Centre. ( a ) End-Paleocene reconstruction of the North Atlantic Igneous Province. Scale bar, 200 km. Adapted with permission from Fig. 7, Saunders et al. [14] , Chemical Geology, v. 241, issues 3–4, Regional uplift associated with continental large igneous provinces: The role of mantle plumes and the lithosphere, 282–318, Elsevier (2007). ( b ) Map of the Carlingford Igneous Centre, showing the Irish National Grid. Cone-sheet intrusions not shown. A thermal aureole of 100–200 m thickness surrounds the igneous centre. Scale bar, 1 km. Intrusions of the adjacent Slieve Gullion Igneous Centre are shown in yellow. Reproduced with permission from the Geological Survey of Ireland 1:100,000 scale bedrock geology map, Geological Survey of Ireland/Government of Ireland (2014). Full size image The Carlingford Igneous Centre (62–60 Myr ago) [22] in County Louth, NE Ireland, lies within the Palaeozoic Longford-Down terrane, an accretionary prism that relates to the closure of the Iapetus Ocean. The crust is considered to be ~\n28–30 km thick in the region and a wide suture zone has been seismically identified at mid-crustal levels beneath Carlingford [23] , [24] . The crust above the suture comprises Ordovician and Silurian metasedimentary rocks, dominantly distal greywackes of greenschist facies metamorphic grade, which were accreted during the closure of Iapetus in the late Silurian [25] . The rocks at and below the suture are poorly understood, known only from wide-angle seismic data and from a limited xenolith suite. Metavolcanic xenoliths from the mid to lower crust are interpreted as volcanic arc material that formed during the closure of the Iapetus Ocean [23] , [25] , as are deep crustal granulite facies xenoliths from central Ireland [24] , [26] . It has therefore been postulated that the entire mid to lower crust in this region is likely to be formed from accreted juvenile arc (or arc-derived) material, and may not include a significantly older crystalline basement [24] , [26] . At the surface, Silurian Longford-Down metasiltstones are unconformably overlain by the Carboniferous Carlingford Limestone [27] , which forms the uppermost ≤200 m of the local bedrock ( Fig. 1b ). A metamorphic aureole surrounds the igneous centre, grading into partially melted diopside and biotite hornfels (Silurian metasedimentary rocks) and coarse wollastonite marble (Carboniferous limestone). Bimodal magmatism at Carlingford is characterized by two main intrusions, a microgranite ring-dyke followed by a gabbro lopolith [27] , [28] , [29] ( Figs 1b and 2 ). The microgranite and gabbro intruded in close temporal succession and show frequent liquid–liquid mixing and mingling textures [28] ( Supplementary Fig. 1 ). These intrusions are crosscut by a swarm of dominantly basaltic (aphyric and plagioclase porphyritic) cone-sheets [30] . Initial work by Halsall [31] suggested three separate cycles of cone-sheet intrusion at the Carlingford Igneous Centre, based on an earlier interpretation of the intrusion sequence [27] , [28] . In light of the currently accepted order of intrusion [29] , we consider the cone-sheets to represent a single intrusion cycle, consistent with recent developments on other cone-sheet swarms in the BPIP, such as those of the Ardnamurchan Igneous Centre [32] . A large gravity and aeromagnetic anomaly has been recognized in the Carlingford region, and is best approximated by a laterally extensive, ~\n10 km thick, mafic intrusion some 2–3 km below the present day land surface [33] , which is ~\n5–6 km below the Palaeogene land surface, when subsequent erosion is considered [34] . This large intrusive body was the feeder for high-level activity at Carlingford, and the adjacent Slieve Gullion Igneous Centre [33] , and implies a significant heat source was available within the upper crust at the time. Full petrological descriptions of the igneous and crustal rocks at Carlingford are provided in Supplementary Note 1 and Supplementary Figs 1,2 . 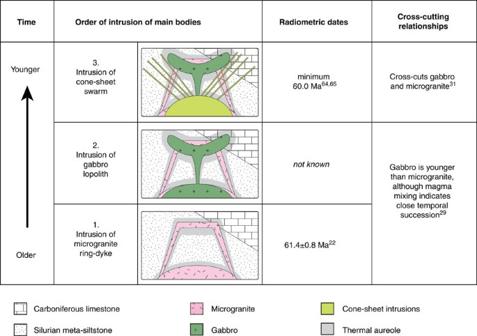Figure 2: Intrusion sequence and age relationships at the Carlingford Igneous Centre. Schematic cross sections are based on field evidence29,31and available radiometric dates22,64,65. Figure 2: Intrusion sequence and age relationships at the Carlingford Igneous Centre. Schematic cross sections are based on field evidence [29] , [31] and available radiometric dates [22] , [64] , [65] . Full size image Here we apply a multifaceted petrological, geochemical, experimental and numerical approach to investigate the likely causes of bimodal magmatism in the BPIP, using the Carlingford Igneous Centre as a case study ( Fig. 1b ). We test current models for the generation of felsic magmas by crustal melting [9] , [11] , and question why felsic magmatism is usually only seen in the early stages of individual BPIP centres [15] , [16] , [19] , [21] . We propose that the potential to produce large volumes of felsic magma by crustal assimilation rapidly decreases during the lifetime of an igneous centre as the local crust becomes progressively more refractory with each intrusion and subsequent crustal melting event. We term this process ‘progressively inhibited crustal assimilation’ (PICA), and the consequent return to mafic magmatism results in a strongly bimodal magma suite. Major and trace elements The gabbro represents the most primitive composition at Carlingford ( Fig. 3a ) and appears to relate to the basalt cone-sheets by fractional crystallization, likely reflecting derivation from a common parent magma ( Fig. 3b–e ; Supplementary Fig. 3 ). A common evolutionary trend for the gabbro and cone-sheet basalt is reinforced by a uniform Zr versus Nb trend, indicating crystal fractionation was a key process ( Fig. 3f ). 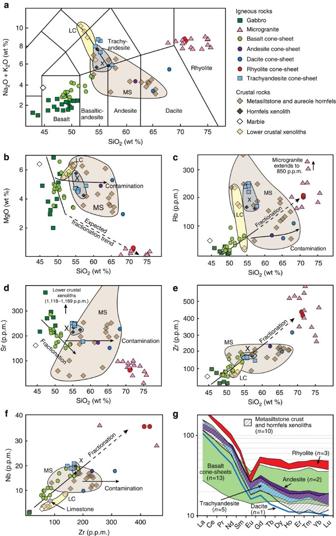Figure 3: Geochemical plots of Carlingford rock compositions. Metasedimentary rock field (MS) includes metasiltstone and aureole hornfels rocks from Carlingford and the nearby Mourne and Slieve Gullion Centres. The hornfels xenoliths (X) are found in close association with the trachyandesite samples in a late cone-sheet intrusion. The lower crust is characterized via new analyses of the xenoliths of Anderson and Oliver23. Limestone is not shown (22% SiO2). Major and trace element data for the gabbro and microgranite from this study (n=4) are combined with published data from refs27,28,31and references therein; however, there are no published data for Nb. Metasiltstone and hornfels samples from this study (n=10) are supplemented with data from refs17,27,31,66,67. (a) Total alkali versus silica diagram. (b) MgO versus SiO2, fractionation trend from Furmanet al.35(c) Rb versus SiO2. (d) Sr versus SiO2. (e), Zr versus SiO2. (f) Zr versus Nb. (g) Chondrite normalized54rare earth element diagram of cone-sheet compositions and Longford-Down metasedimentary rocks. Figure 3: Geochemical plots of Carlingford rock compositions. Metasedimentary rock field (MS) includes metasiltstone and aureole hornfels rocks from Carlingford and the nearby Mourne and Slieve Gullion Centres. The hornfels xenoliths ( X ) are found in close association with the trachyandesite samples in a late cone-sheet intrusion. The lower crust is characterized via new analyses of the xenoliths of Anderson and Oliver [23] . Limestone is not shown (22% SiO 2 ). Major and trace element data for the gabbro and microgranite from this study ( n =4) are combined with published data from refs 27 , 28 , 31 and references therein; however, there are no published data for Nb. Metasiltstone and hornfels samples from this study ( n =10) are supplemented with data from refs 17 , 27 , 31 , 66 , 67 . ( a ) Total alkali versus silica diagram. ( b ) MgO versus SiO 2 , fractionation trend from Furman et al. [35] ( c ) Rb versus SiO 2 . ( d ) Sr versus SiO 2 . ( e ), Zr versus SiO 2 . ( f ) Zr versus Nb. ( g ) Chondrite normalized [54] rare earth element diagram of cone-sheet compositions and Longford-Down metasedimentary rocks. Full size image Ten cone-sheet samples are more evolved than the rest of the cone-sheet suite ( n =15) and classify as andesite, trachyandesite, dacite and rhyolite ( Fig. 3a ). Notably, the trachyandesites were collected close to large (>1 m), high-K 2 O hornfels xenoliths (data field ‘X’ in Fig. 3 ). These intermediate cone-sheet samples all maintain elevated MgO values and resemble the composition of the metasiltstone aureole and hornfels xenoliths instead of closed-system fractional crystallization trends [35] ( Fig. 3b ). They also plot in or near the crustal fields for both incompatible and compatible trace elements ( Fig. 3c–e , Supplementary Fig. 3 ). While the andesite and dacite samples shift towards higher Zr at constant Nb concentrations and reach values similar to those of the metasiltstone country rocks, the trachyandesites echo the hornfels xenoliths’ trace element characteristics. The REE patterns of the andesite, dacite and trachyandesite confirm a strong crustal influence on their petrogenesis ( Fig. 3g ). To test the hypothesis that the trachyandesite ‘magma’ is actually derived by melting of the adjacent xenolith(s), least-squares mixing analysis was used to produce a best-fit binary mixing ratio for basalt CS4E and hornfels xenolith C-SB1. Major element calculations suggest the trachyandesite is 99% hornfels derived, while the trace element model gives a value of 88%, because the trachyandesite is enriched in Sr and Rb relative to both the basalt and the hornfels. This disparity between major and trace element mixing proportions is explained by the production and loss of an enriched partial melt from the hornfels (due to melting of feldspar and biotite [36] ). Many of the hornfels xenoliths show partial melting textures ( Fig. 4a,b ), consistent with the notion that the trachyandesite is actually a crustal melt, rather than a mantle-derived magma. 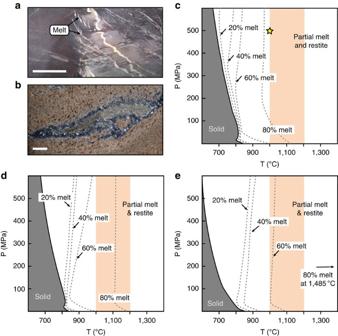Figure 4: Field and thermochemical evidence for partial melting in Carlingford metasedimentary crust. (a) Hand specimen of a hornfels xenolith with merging melt pockets that once formed a melt network. Scale bar, 5 mm. (b) Thin section image of former melt pocket in hornfels xenolith. Scale bar, 250 μm. (c–e) Theoretical melt volume isopleth models were calculated for Longford-Down metasedimentary samples of increasing metamorphic grade; (c) pristine metasiltstone, (d) aureole hornfels and (e) hornfels xenolith. Yellow star incmarks the position of our melting experiment. This experiment showed near-complete melting (95–99%) of pristine metasiltstone. The slight mismatch with the model most likely reflects heterogeneities in water content. The vertical orange bar indicates the magmatic temperature range. Figure 4: Field and thermochemical evidence for partial melting in Carlingford metasedimentary crust. ( a ) Hand specimen of a hornfels xenolith with merging melt pockets that once formed a melt network. Scale bar, 5 mm. ( b ) Thin section image of former melt pocket in hornfels xenolith. Scale bar, 250 μm. ( c – e ) Theoretical melt volume isopleth models were calculated for Longford-Down metasedimentary samples of increasing metamorphic grade; ( c ) pristine metasiltstone, ( d ) aureole hornfels and ( e ) hornfels xenolith. Yellow star in c marks the position of our melting experiment. This experiment showed near-complete melting (95–99%) of pristine metasiltstone. The slight mismatch with the model most likely reflects heterogeneities in water content. The vertical orange bar indicates the magmatic temperature range. Full size image The rhyolite cone-sheet samples lie on the projected gabbro–basalt fractionation trend for all elements ( Fig. 3b–e ), implying they are the products of fractionation from this, or a similar, basaltic parent. The early microgranite, in contrast, was considered to be entirely crustal in origin by previous authors [28] , [31] . The microgranite is indeed relatively enriched in heavy REEs, with highly variable concentrations of incompatible elements such as Rb and Zr, and deviates significantly from an expected magmatic fractionation trend. These data infer a significant crustal influence on the microgranite formation and we argue that large volumes of incompatible element-enriched partial melts of the metasiltstones [37] have contributed to its genesis ( Fig. 3c,e ; Supplementary Fig. 3 ). The interaction of both mafic mantle and felsic crustal melts is consistent with frequent mingling and mixing textures recorded at, for example, Barnavave and Slievenaglogh [28] (See Supplementary Fig. 1 ). Experimental petrology and thermodynamic modelling To test the chemical influences of the local crust inferred from our major and trace element data, we performed a high-pressure, high-temperature melting experiment and carried out thermodynamic modelling on the Silurian country rock. A sample of metasiltstone produced >95% melt when heated to 1,000 °C at 500 MPa for 1 h in a piston cylinder apparatus, emphasizing its advanced fusibility at magmatic temperatures and at short timescales (hours to days). Melt volume isopleths for three crustal samples, that reflect the various metamorphic grades of the Carlingford aureole, were modelled using Perple_X [38] ( Fig. 4c–e ). At 200 MPa and 780 °C, the models indicate that pristine Longford-Down metasiltstone will generate 30% melt. This pressure represents a depth of ~\n6–7 km, consistent with the top of the regional gravity anomaly and the hypothesized location of the feeder chamber for the Carlingford Igneous Complex [27] , [33] , [34] . Melt volumes of ~\n25% are generally considered the threshold for a free-moving melt system [39] , [40] , although permeable melt networks may be maintained at ≤5% melt [40] . These results suggest partial melting can occur quickly and that melts were transported over a wide aureole zone, consistent with the widespread occurrence of rheomorphic pyroxene hornfels in the Carlingford metamorphic aureole and with published models of the thermal effects of basaltic intrusions on crustal rocks [9] . The aureole hornfels and the high-K 2 O hornfels xenoliths both melt to a lesser degree than the pristine metasiltstone, with 30% melt reached at 835 °C and 865 °C, respectively, documenting a reduction in the crustal melt-generation capacity with successive melt-loss events ( Fig. 4 ). Radiogenic isotope geochemistry Sr, Nd and Pb isotopes reveal that all igneous samples from Carlingford deviate from mantle values and require various amounts of crustal addition ( Fig. 5a–c ). None of the data available from the lower crustal xenoliths [23] , which are likely to be representative of the rocks present at lower crustal depths [24] , [26] , are sufficiently radiogenic to produce the observed magmatic isotope signatures through assimilation. The Carlingford Limestone, in turn, occupies a higher structural level than the majority of the igneous intrusions, and as such, it cannot have interacted with the Carlingford magmas in a major way. We must conclude that the Longford-Down mid to upper crustal metasedimentary rocks are the primary isotopic influence recorded at Carlingford, which is supported by the geophysical evidence for a large volume of mafic intrusives at shallow levels in the crust beneath Carlingford [33] . Although there may have been a degree of lower crustal contamination, it is impossible to detect due to the subsequent interaction with the considerably more radiogenic Longford-Down metasedimentary suite. 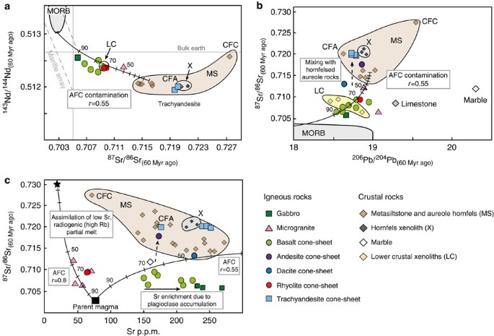Figure 5: Radiogenic isotope plots for the Carlingford Igneous Centre. Parental magma values from refs21,60,61. (a)87Sr/86Sr versus143Nd/144Nd. (b)206Pb/204Pb versus87Sr/86Sr. (c) Sr p.p.m. versus87Sr/86Sr.cincludes data from this study combined with published data for gabbro (n=1)68, microgranite (n=2)68,69and metasedimentary crust (n=11)17,67,70. AFC models for gabbro and basalt ina–cuse a metasiltstone hornfels (MSC-2) from the nearby Mourne Intrusive Centre and anr-value of 0.55. Sr-enrichment incindicates high plagioclase content in both porphyritic basalt cone-sheets and gabbro (see also positive Eu anomaly for the gabbro inSupplementary Fig. 3). CFC, Carlingford pristine crust, CFA, Carlingford aureole hornfels. Inc, assimilation of a crustal partial melt (black star) is modelled using a hypothetical end-member composition (87Sr/86Sr=0.73000, Sr=10 p.p.m.) and anr-value of 0.8. Figure 5: Radiogenic isotope plots for the Carlingford Igneous Centre. Parental magma values from refs 21 , 60 , 61 . ( a ) 87 Sr/ 86 Sr versus 143 Nd/ 144 Nd. ( b ) 206 Pb/ 204 Pb versus 87 Sr/ 86 Sr. ( c ) Sr p.p.m. versus 87 Sr/ 86 Sr. c includes data from this study combined with published data for gabbro ( n =1) [68] , microgranite ( n =2) [68] , [69] and metasedimentary crust ( n =11) [17] , [67] , [70] . AFC models for gabbro and basalt in a – c use a metasiltstone hornfels (MSC-2) from the nearby Mourne Intrusive Centre and an r -value of 0.55. Sr-enrichment in c indicates high plagioclase content in both porphyritic basalt cone-sheets and gabbro (see also positive Eu anomaly for the gabbro in Supplementary Fig. 3 ). CFC, Carlingford pristine crust, CFA, Carlingford aureole hornfels. In c , assimilation of a crustal partial melt (black star) is modelled using a hypothetical end-member composition ( 87 Sr/ 86 Sr=0.73000, Sr=10 p.p.m.) and an r -value of 0.8. Full size image The gabbros and cone-sheet basalts define a trend that is compatible with assimilation of metasiltstone during fractional crystallization (AFC) [41] ( Fig. 5a,b ), while the cone-sheet andesite and dacite samples plot off this main trend and require a two-step crustal assimilation origin. Initial AFC-type processes were followed by bulk mixing of the already contaminated magma with crustal (partial) melts [42] , explaining their strong major and trace element similarity to the crustal rocks. In stark contrast, cone-sheet rhyolites have similar isotopic ratios to the basalts, implying a late-stage cessation of basalt–crust interaction and closed-system fractionation of basalt to rhyolite during the final stages of magmatic activity at the Carlingford Igneous Centre ( Figs 3 , 5a,b ). The trachyandesites, in turn, have isotope compositions that are virtually identical to the hornfels xenoliths ( Fig. 5 ). These data strongly support the results of the major and trace element mixing modelling and imply that the trachyandesites are an ‘S-type’ melt that formed when the continued flow of hot basalt (~\n1,100 °C) around hornfels xenoliths during cone-sheet emplacement supplied the necessary heat for large degrees of partial fusion of the hornfels xenoliths (≥865 °C) ( Fig. 4 ). The large volume early microgranites cannot be a whole rock or high-degree partial melt of metasiltstone, as proposed by previous authors [28] , [31] , as their Sr isotope compositions are not sufficiently radiogenic. Rather, they are consistent with the formation from enriched crustal partial melts combining with less-radiogenic, mantle-derived magma(s). Considering that the restitic aureole hornfels at Carlingford (CFA in Fig. 5 ) is less radiogenic and has higher Sr concentrations than its metasiltstone protolith (CFC in Fig. 5 ), the metasiltstone must have released a water-rich, radiogenic (Rb-rich), low-Sr partial melt during biotite and chlorite breakdown [9] , [36] ( Fig. 5c ). Such melts can be produced in high volumes by heating the metasiltstone above ~\n750 °C ( Fig. 4c ). Incorporation of large amounts of enriched partial melts of this type would result in rapid differentiation to felsic compositions due to high rates of crustal incorporation [43] (for example, r =0.8, Fig. 5c ). Plagioclase microanalysis To test for progressive changes in the degree of magma–crust interaction, we analysed successive zones in representative plagioclase phenocrysts from a porphyritic basalt cone-sheet at Slate Rock for major elements (170 analyses) and in situ Sr-isotope ratios (9 analyses) ( Fig. 6a–c ). All crystals display a similar anorthite zoning pattern, recording high anorthite cores and an overall decrease in anorthite values towards the rims, albeit with some internal resorption surfaces ( Fig. 6a–c ). Crystal cores show elevated 87 Sr/ 86 Sr ratios when compared with mantle values, indicating growth from contaminated magma. The 87 Sr/ 86 Sr values of subsequent rims fluctuate notably with distance from the core, and are unlikely to reflect simple AFC-style crystallization [44] , but rather suggest interaction with magmas of variable isotopic composition. 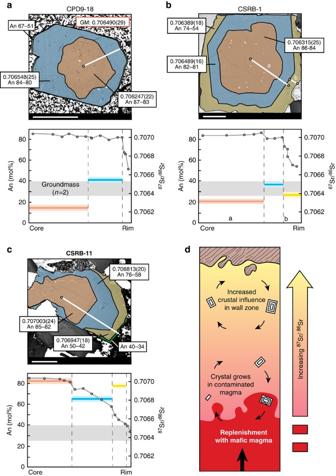Figure 6:In situcrystal isotope stratigraphy of representative plagioclase crystals from late porphyritic basalt cone-sheets. (a–c) Colour-coded Backscattered electron (BSE) images show crystal zones and microprobe traverse paths. White scale bars are 500 μm long in each case. Graphs below BSE images show microdrilled strontium isotope ratios (coloured bars, lighter areas represent two s.e.) and microprobe traverses of An values (grey circles). Grey horizontal bars indicate the range of groundmass isotope values (n=2) from in situ (seeaandSupplementary Table 1) and bulk separate analyses (seeSupplementary Data 1). Vertical grey dashed lines delineate crystal zone boundaries. (d) Schematic cross section through the Carlingford cone-sheet magma chamber. The chamber is likely to have had an isotopic gradient, with higher crustal input towards the walls and the roof. Crystals CPD9-18 (a) and CSRB-1 (b) record progressive contamination (see cores and rim 1) while CSRB-11 (c) is likely to have grown near the chamber edge. Notably, CSRB-1 and CSRB-11 are from the same sample, indicating crystal populations were thoroughly mixed during transport and dyke emplacement. Figure 6: In situ crystal isotope stratigraphy of representative plagioclase crystals from late porphyritic basalt cone-sheets. ( a – c ) Colour-coded Backscattered electron (BSE) images show crystal zones and microprobe traverse paths. White scale bars are 500 μm long in each case. Graphs below BSE images show microdrilled strontium isotope ratios (coloured bars, lighter areas represent two s.e.) and microprobe traverses of An values (grey circles). Grey horizontal bars indicate the range of groundmass isotope values ( n =2) from in situ (see a and Supplementary Table 1 ) and bulk separate analyses (see Supplementary Data 1 ). Vertical grey dashed lines delineate crystal zone boundaries. ( d ) Schematic cross section through the Carlingford cone-sheet magma chamber. The chamber is likely to have had an isotopic gradient, with higher crustal input towards the walls and the roof. Crystals CPD9-18 ( a ) and CSRB-1 ( b ) record progressive contamination (see cores and rim 1) while CSRB-11 ( c ) is likely to have grown near the chamber edge. Notably, CSRB-1 and CSRB-11 are from the same sample, indicating crystal populations were thoroughly mixed during transport and dyke emplacement. Full size image In an effort to constrain the depth of contamination, we performed mineral melt equilibrium thermobarometry [45] , [46] on cone-sheet plagioclase crystals to gauge the approximate pressure (depth) at which these crystals grew. Despite the large errors inherent to the method, results of 180–270 MPa±247 MPa (equivalent to depths of 6–9 km±8 km), imply crystallization is likely to have occurred in the mid to upper crust, placing the feeder reservoir to the Carlingford Igneous Centre within the metasiltstone rocks of the Longford-Down massif. Significantly, these results are complemented by down-dip projections of the cone-sheets, which suggest uppermost magma storage at a depth of ~\n6 km i [31] , [34] , while geophysical models indicate the top of an extensive (~\n10 km thick) mafic pluton at ~\n5–6 km i depth [33] , [34] (where km i indicates initial depth below the Palaeogene land surface, prior to erosion). Full discussion of the thermobarometry results and errors are provided in Supplementary Note 2 . The Sr isotope compositions of the groundmass and those of rims 1 and 2 in crystals CPD9-18 and CSRB-1 ( Fig. 6a,b ), are very similar (0.7065±0.0002), supporting a strong genetic link and indicating the rims are in equilibrium with the surrounding groundmass. In contrast, the cores of crystals CPD9-18 and CSRB-1 have less-radiogenic Sr isotope ratios than the groundmass, indicating they have grown from a less evolved, less contaminated magma. CSRB-11’s core has a higher Sr isotope ratio than any of the other analysed crystals (core or rim), but has the same anorthite range as the rest of the cores, indicating it grew from a more contaminated magma but with a similar major element composition (for example, near the walls or roof of the chamber). The common pattern of anorthite values for all crystals analysed by electron microprobe (EMP) implies they all grew in the same magma system, which appears to have contained an isotopic gradient, likely due to increased contamination near the roof/walls combined with magma replenishment at the base of the chamber. Convection is expected in such a chamber and can explain the variation in isotopic compositions observed between the cores and subsequent rims in the three in situ plagioclase examples ( Fig. 6d ). Repeated replenishment would account for the resorption surfaces seen in many of the crystals and implies that isotopic gradients were maintained for some time. Such replenishments would swiftly exhaust country rock fertility through successive partial melting events, so crustal contamination would become progressively less important as time progressed, consistent with our thermodynamic models ( Fig. 4c–e ) and the formation of late rhyolitic cone-sheets by fractional crystallization alone. Our combined whole-rock and in situ crystal data imply the Longford-Down metasiltstone was the overwhelming crustal influence on the Carlingford magmas, although additional, less radiogenic, lower crustal input cannot be fully excluded. Initial intrusion of a large volume of mafic magma at mid to upper crustal levels (~\n5–6 km) is supported by structural studies [27] , [31] , [34] , geophysical observations [33] and the presented thermobarometric models (see also Supplementary Note 2 ). This considerable magma reservoir heated the surrounding crust and resulted in intense partial melting defined by the 750–800 °C isotherm and a progressively wider contact aureole ( Figs 1b , 4 ). Large-scale incorporation of partial melts by ascending mafic magmas allowed rapid differentiation by AFC, forming the microgranite. Trace element variability in the microgranite implies that the partial melt was enriched in incompatible elements, including Rb and Zr. These earliest ‘low-temperature’ crustal melts were quickly exhausted and subsequent melt-extraction events (driven by successive magmatic replenishments) progressively lowered the fertility of the metasiltstone, until only a refractory hornfels restite remained. Our melting experiment and thermodynamic models for the aureole rocks replicate these physical and temporal changes and define the thresholds of achievable anatexis in the Carlingford system ( Fig. 4c–e ). The net result of successive melt-extraction events is to progressively lower crustal melt volumes, which will also become increasingly less radiogenic in composition [36] . Extensive microgranite formation was thus limited to the early stages of magmatism at the Carlingford Igneous Centre, when enriched metasiltstone partial melts were formed and accelerated differentiation was possible. Subsequent replenishment(s) of the magma system resulted in progressively more restricted assimilation of increasingly refractory compositions, forming mildly contaminated gabbros and basalts (see Figs 2 , 3 ). Intermediate igneous rocks are exceptionally rare at Carlingford, forming <1% of the total volume of igneous rocks and there is no evidence that large volumes of intermediate magma were ever generated. Localized trachyandesite compositions are shown to be pure crustal melts, rather than mantle-derived magmas, and were only formed locally around xenoliths, during transport in cone-sheets. The andesite and dacites formed in a different manner, when xenolith or wall rock melts were ultimately mixed into already contaminated basaltic magmas as they flowed during emplacement, a process known as assimilation during turbulent ascent [47] . Finally, the cone-sheet rhyolites, the most evolved compositions from the late cone-sheet suite, are the products of fractionation of a basaltic parent, as indicated by their major and trace element trends and isotopic composition ( Figs 3 , 5 ). These rocks imply that widespread magma–crust interaction was no longer a major differentiation process during the final stages of activity at Carlingford, reflecting the refractory nature of the crust by this point in time. Our results are consistent with published thermodynamic, numerical and analogue models [9] , [10] , [11] , [12] , which show that repeated basaltic intrusion can cause bimodal magmatism due to crustal melting and rapid differentiation. However, our study shows that continental crust has a finite ability to produce large volumes of fertile partial melt and quickly becomes refractory. These findings mean that, after a certain point (determined by the composition of the crust), repeated basaltic intrusions cannot increase the degree of crustal partial melting any further. Instead, progressively lower volumes of increasingly less fertile crustal melts are produced ( Fig. 4c–e ), which ultimately results in a return to mafic magmatism. Contrary to most previous models [10] , [12] , which predict increasing volumes of felsic magmas with prolonged crustal heating, our data from Carlingford suggest that bimodal magmatism is the product of a decline in assimilation-driven differentiation due to a systematic reduction in the crustal fertility with successive intrusion events, a process we term progressively inhibited crustal assimilation (PICA). Only the generation of new magma pathways and lateral exploitation of ‘fresh’ crust would result in a resurgence in felsic magmatism. While we demonstrate PICA for fertile mica and chlorite-rich metasedimentary compositions at Carlingford, this process would also be effective in more difficult to melt rocks, such as gneiss or basalt, where partial melt-extraction events are very effective at causing the crust to quickly become even more refractory than in our case study [36] . For example, large-scale partial melting of Lewisian gneiss is documented in the early stages of the Rum and Skye central complexes, where early felsic magmas show a strong crustal component and are typically followed by less contaminated mafic compositions [15] , [16] , [21] . Likewise, assimilation of partial melts from hydrated basaltic crust has been shown as a source for Icelandic rhyolites [48] . The PICA process likely also operated on a large scale at Mull, where Centre 1 shows extremely radiogenic Sr-isotope signatures indicating the incorporation of large volumes of radiogenic crustal melt, while Centre 2, which crosscuts Centre 1, shows a greater proportion of mafic rocks and a much more restricted (that is, less crustal) isotope geochemistry [19] . Together, this evidence indicates that PICA could be a significant cause of bimodal mafic–felsic magmatism throughout both the BPIP and the NAIP. Magma–crust interaction has also been widely recognized as an important contributor to felsic magma generation in other continental flood basalt provinces (for example, Karoo, Paraná-Etendeka, Deccan, Yemen) [13] and a decline in crustal fertility with time has been recently noted at Yellowstone [49] , indicating that the PICA process may also be applicable to a range of other volcanic regions. Sample selection and preparation All raw data and sample locations are presented in Supplementary Table 1 , Supplementary Data 1–3 . Representative samples of the main lithologies exposed at the Carlingford Igneous Centre were collected (total n =47), although the cone-sheet swarm was sampled in more detail ( n =27), as sampling included traverses through individual sheets ( Supplementary Data 1,2 ). Samples were sliced and weathered edges removed. The samples were crushed in a jaw crusher and powdered in a Tema T100 tungsten carbide disc mill at the Department of Geology, Trinity College Dublin. All powders were analysed for major and trace elements and a selected sample sets were further analysed for rare earth elements and strontium, neodymium and lead isotopes. X-Ray fluorescence Whole rock and groundmass samples were analysed for major element oxides and trace element concentrations by XRF at GEOMAR Research Centre, Kiel, Germany. Samples were analysed on fused beads using a Philips PW1480 spectrometer and an Rh tube. Calibration was performed using international geological reference samples [50] . CO 2 and H 2 O contents were measured by IR photometry using a Rosemount CSA 5003 at GEOMAR. Major element data had initial totals ranging from 99.00–100.82% (See Supplementary Data 1,2 ) and were corrected for loss on ignition and normalized to 100% for plotting and modelling. Additional XRF analyses on gabbros C4, C7 ; microgranites LWG1, LWG2 ; rhyolites 284-8c, 288-8a ; metasiltstone Silt1 ; lower crustal metasedimentary rocks BWA, BWB, BWC, BWD and Carboniferous carbonates Limestone 1, Marble 1 were carried at the University of St Andrews, Scotland. Samples were analysed using fused beads on a Spectro X-Lab EDP XRF. All analyses were performed with an Rh tube and calibration was performed using international geological reference samples [51] . Major element data had initial totals ranging from 99.20–100.02% (See Supplementary Data 1,2 ) and were also corrected for loss on ignition and normalized to 100% for plotting. Inductively coupled plasma mass spectrometry Rare earth elements and U, Th and Pb concentrations were determined by ICP-MS at the Scottish Universities Environmental Research Centre (SUERC), East Kilbride, Scotland, using a VG Elemental PQ2 plus ICP-MS fitted with a Meinhard nebulizer and a water-cooled glass Scott double pass spray chamber [52] (see Supplementary Data 1,2 ). Analyses of geological reference standard BCR-1 throughout this study ( n =36) yielded an average s.d. of 0.38 p.p.m. over mean values of 14 rare earth elements when compared with published values [53] . Values were chondrite normalized [54] before plotting. Experimental petrology A 1 cm long, 3 mm diameter cylindrical rock sample of Longford-Down metasiltstone [SILT1] was heated for 1 h at 1,000 °C and at a pressure of 500 MPa, using an end-loaded piston cylinder apparatus. The platinum capsule containing the sample was positioned into a 19.1 mm NaCl-crushable alumina-pyrex assembly. The assembly was cold-pressurized to 500 MPa and was maintained at a constant pressure for the duration of the experiment and during quench. The temperature was measured using factory-calibrated C-type (W 95 Re 5 –W 74 Re 26 ) thermocouples with an uncertainty of ±3 °C. After quenching, the sample was mounted in resin and imaged using a field emission scanning electron microscope (JEOL FE-SEM 6500F equipped with an energy dispersive microanalysis system). Both facilities are at the HP-HT Laboratory of Experimental Volcanology and Geophysics at the Istituto Nazionale di Geofisica e Vulcanologia (INGV) Rome. Radiogenic isotope geochemistry Selected samples were analysed for strontium, neodymium and lead isotope ratios at the Scottish Universities Environmental Research Centre (SUERC) (See Supplementary Data 1,2 ). Sr was separated using standard cation exchange techniques with a single pass through Bio-Rad AG50W-X-12 resin. The samples were loaded on single Ta filaments with 1 M phosphoric acid. Isotope ratios were measured on a VG Sector 54–30 thermal ionization mass spectrometer in dynamic multi-collection mode and corrected for instrumental mass fractionation using an exponential law and 87 Sr/ 88 Sr=0.1194. Total procedure blanks were <300 pg. The internal laboratory Sr Standard (NBS987) was analysed as 0.710254±18 (2 σ ) for the duration of this study. Rare earth elements were collected by cation exchange from the same samples as the Sr fraction. Nd was separated by standard anion exchange chemistry and analysed using a VG Sector 54–30 thermal ionization mass spectrometer. The internal laboratory Nd Standard (J&M) was analysed as 0.511504±9 (2 σ ) for the duration of this study. Lead chemistry was performed separately and was analysed by a Micromass Isoprobe MC-ICP-MS, using the techniques detailed by Ellam [55] . Total procedural blank was 352 pg. Measurements of NIST SRM981 were used to correct the data. Uncorrected NIST SRM981 gave values of 206 Pb/ 204 Pb=16.939±31, 207 Pb/ 204 Pb=15.497±19, 208 Pb/ 204 Pb=36.719±64 (2 s.d., n =12). Plagioclase microanalysis Samples CPD9 and CSRB are representative of the range of phenocryst compositional variations observed within the cone-sheet porphyritic basalt. Zoned phenocrysts were identified using a petrological microscope and were then imaged using backscattered electron microscopy, before being systematically investigated through spot analyses ( Supplementary Data 3 ). Feldspar major element compositions were determined using a JEOL JCXA 733 EMP at the University of St Andrews, Scotland. Analytical conditions included an acceleration voltage of 15 kV, a beam current of 8–20 nA and counting times between 20 and 60 s on peaks. A rastered beam was used ( ca . 12 μm 2 ) and calibration was performed using natural and synthetic minerals as standards. Backscattered electron images of feldspars were also collected. Microdrilling for Sr isotope ratios of individual feldspar zones was carried out using a Merchantek/New Wave Micromill at the University of Durham, UK ( Supplementary Table 1 ). Zones were identified both optically and in backscattered electron images of polished thick sections. The milling technique and subsequent microchemistry are described in more detail in Charlier et al. [56] The samples yielded between 1.9 and 13 ng of Sr per zone drilled and all samples were analysed successfully for 87 Sr/ 86 Sr isotope ratios. The internal laboratory Sr Standard (NBS987) was analysed as 0.710259±12 (2 s.d.) for the period of the study. Plagioclase-melt thermobarometry The H 2 O-calibrated plagioclase-melt thermobarometer of Putirka [45] , [46] was used to calculate plagioclase-melt equilibria and estimate the pressure (depth) of crystallization of the cone-sheet plagioclase phenocrysts. Melt compositions are represented by groundmass separate GM1 that was hand-picked from whole rock crush, and analysed for major elements by XRF at GEOMAR Research Centre, Kiel, Germany (see above). This melt value was compared with 170 plagioclase EMP spot analyses, representing core to rim traverses of phenocrysts. The thermobarometer is particularly sensitive to water content and a H 2 O value of 1.4% was used, as determined by IR photometry on GM1. The anorthite-albite partition coefficient ratio (Kd [An–Ab] ) is recommended as an equilibrium test for plagioclase-melt thermobarometry and hence, only plagioclase compositions that lay within Kd [An–Ab] values of 0.27±0.11 (considering T >1,050 °C) were accepted as reliable [46] . The standard errors of estimate for this thermobarometer are given as±36 °C and±247 MPa [46] . Partial melting modelling The Perple_X’07 software package [38] was used to model theoretical isopleths of melt volume for three end members; metasiltstone [SILT1], aureole hornfels [C-LD1] and hornfels xenolith material [C-SB2]. Models were performed in the NCKFMMnASHTi system using the Holland and Powell internally consistent thermodynamic data set [57] . Haplogranitic melt [58] , [59] was used as the solution model (available from the solute_08.dat datafile of Perple_X). Water was treated as an undersaturated phase, making these theoretical models directly comparable to the melting experiment. The models suggest that at 200 MPa (~\n6–7 km depth) and ~\n760 °C, pristine regional crust [SILT1] begins to partially melt and is 60% molten by 810 °C, which indicates rapid melt production over a very narrow temperature interval ( Fig. 4c ). Hornfels [C-LD1], from within the metamorphic aureole, begins melting at a similar temperature, although the extent of melting does not increase as rapidly as SILT1. Nevertheless, 60% melt is reached by 875 °C ( Fig. 4d ). The xenolith hornfels material [C-SB2] begins with low degrees of melting at ~\n680 °C, but does not progress to 60% melt until ~\n1,010 °C ( Fig. 4e ). Both these hornfels samples show evidence for partial melt loss (for example, Fig. 4a,b ) and are thus a restite with respect to pristine metasiltstone crustal compositions (for example, SILT1). Radiogenic isotope modelling Using a typical Atlantic MORB basalt [60] , [61] and the local metasiltstone as end members, geochemical models for both AFC [41] and bulk mixing [42] were calculated. MORB values were used as the starting composition because a depleted mantle source is considered typical for the province [61] , [62] . AFC modelling employed the AFC.isotopes spreadsheet of J. Entenmann (University of Göttingen), which uses published models and equations [41] , [63] . Modelling was run over a range of r -values, to consider the effect of various amounts of assimilation. The r -value represents the ratio of AFC, with high r -values representing high levels of assimilation [43] . Mantle Sr and Nd end members are after Saunders et al. [60] and Pb end members were taken from Ellam and Stuart [61] and Meyer [21] . How to cite this article : Meade, F. C. et al. Bimodal magmatism produced by progressively inhibited crustal assimilation. Nat. Commun. 5:4199 doi: 10.1038/ncomms5199 (2014).